Detection of graphene domains and defects using liquid crystals The direct observation of the domain size and defect distribution in a graphene film is important for the development of electronic applications involving graphene. Here we report a promising method for observing graphene domains grown by chemical vapour deposition. The unavoidable development of crack or pinhole defects during the growth and transfer processes is visualized using a liquid crystal layer. Liquid crystal molecules align anisotropically with respect to the graphene domains and exhibit distinct birefringence properties that can be used to image the graphene domains. This approach is useful for visualizing the crack distributions and their generation process in graphene films under external strain. This type of simple observation method provides an effective route to evaluating the quality and reliability of graphene sheets for use in various electronic devices. The recent production of large-area high-quality graphene (Gr.) films using chemical vapour deposition (CVD) techniques [1] and the ability to transfer such films onto a variety of large-area substrates suggest that these films may be useful as transparent conductive films in a variety of optoelectronic devices [2] , [3] ; however, several types of defects, such as pinholes [4] , [5] , [6] , [7] , [8] , grain boundaries [4] , [9] , [10] and cracks [11] , can form during the CVD growth process or during the transfer step [11] , [12] to a target substrate. These defects degrade the electrical [13] , [14] and mechanical performances of the Gr. [15] , which limits the quality of Gr. available for practical applications. Knowledge of the mechanisms by which defects are generated in Gr. under high strain [5] , [16] is important for the use of Gr. in flexible and stretchable electronic devices. The electrical properties of Gr. grown using CVD methods depend strongly on the domain size and distribution. A variety of methods have been examined for directly observing the defects and domains in Gr. and for understanding the mechanisms by which the defects are generated. For example, microscopy tools, such as transmission electron microscopy [4] , [5] , [6] , [8] , [9] , [10] , atomic force microscopy, and scanning tunneling microscopy [7] , have been used to observe the grain boundaries and defects in Gr. films. These methods have several drawbacks, such as the requirement for complicated sample preparation, time delays, and a limited observation area. Recently, Kim et al. [17] reported an effective method for visualizing the domains and grain boundaries in Gr. films using the properties of liquid crystal (LC) molecules, which align anisotropically along the Gr. domain orientations. Kim et al. [17] suggested that Gr. domains form in alignment with the underlying Cu substrate domains. Although this observation method offered unique advantages in terms of rapid imaging and the ability to identify domains in a large-area Gr. film without complicated sample preparation processes, observation of the defect generation process in a Gr. film under strain remained challenging. The strong correlation between the Gr. and Cu domains was contrary to previous reports that Gr. domains can form across the grain boundaries of the underlying Cu substrate. In this paper, we present an effective method for visualizing and identifying the distributions of domains and defects in Gr., including pinhole and crack generated during the growth and transfer processes. The defects and crack propagation in Gr. were visualized by observing phase transitions in an LC mixture due to the interactions of each constituent molecule of the LC mixture with an underlying polydimethylsiloxane (PDMS) substrate. We also suggest that the alignment of the LC molecules over a Gr. film was more strongly correlated with the domain size in Gr. than with the domain size in the underlying Cu substrate. Anisotropic alignment of LC Several types of Gr. sheet with different domain sizes between 5 μm and 100 μm were synthesized using a controlled CVD growth method and were directly compared. The formation of Gr. nucleation seeds was suppressed by reducing the CH 4 flow rate and by controlling the H 2 annealing time ( Supplementary Figs 1,2 and Methods ) [1] , [18] , [19] , [20] , [21] , [22] , [23] . The exact domain sizes in each Gr. sample were determined by interrupting the growth process just before the film had been completely formed. The interconnections between the Gr. domains were, therefore, incomplete and the incomplete Gr. film was printed onto a glass substrate using a standard wet transfer method involving a poly(methyl methacrylate) (PMMA)-supporting film [11] , [12] , [24] . Scanning electron microscopy images and Raman spectra clearly revealed the formation of Gr. sheets with a uniform domain size distribution ( Fig. 1a and Supplementary Figs 3–5 ) [23] . In particular, selected area electron diffraction mapping patterns indicated that the large Gr. domains formed a single crystalline lattice structure ( Supplementary Fig. 6 ). A 0.5 μl droplet of the LC mixture A, which had a clearing point of 80°C, was placed on the Gr. sheets with incomplete grain connections. The droplet was then covered with a thin glass substrate (5 × 5 mm) coated with a uniaxially rubbed planar alignment layer that improved the birefringence image quality ( Fig. 1b and Supplementary Figs 7,8 and Note 1 ). The LC molecules aligned themselves uniformly along the direction, in which the cover glass had been rubbed, on the glass region that was not covered with the Gr. sheets due to weak anchoring on the glass surface; however, the nematic LCs aligned on the Gr. surface such that the orientations of each domain differed, thereby clearly delineating each domain. The PMMA residue, left by the transfer process on the Gr. layer, exhibited different luminance properties compared with the surrounding area, indicating a distinct alignment of the LC molecules relative to the region coated with pure Gr. Although the PMMA residue domains appeared as defects, they did not influence the overall LC alignment on the Gr. domains due to their relative sparsity ( Supplementary Figs 9,10 and Notes 2,3 ). An LC is a self-assembled, birefringent, dielectric, elastic continuum, and its anisotropic direction of alignment is determined and confined by an anisotropic boundary domain. If the anchoring energy and the boundary domain are large enough to accommodate the elastic energy of the LC, the LC molecules preferentially align according to the anisotropy of each domain, thereby permitting visualization of the exact shape of each domain [25] ( Supplementary Fig. 11 ). It is not clear how a Gr. domain with six-fold symmetry would produce a uniformly anisotropic LC alignment. Although LC alignment is known to rely on the π-stacking interactions between Gr. and LC molecules [17] , [18] , [26] , this effect does not explain the preference of one easy axis over the other two. Further study is needed to understand the origin of LC alignment on Gr. 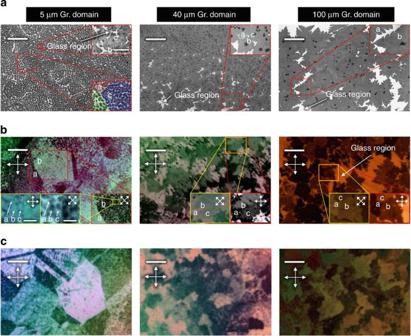Figure 1: Graphene domain size and LC alignment. (a) Scanning electron microscopy images of graphene (Gr.) synthesized through an incomplete growth process on a Cu foil, then transferred onto a glass substrate (The insets show magnified images of a single domain of Gr. The inset in the bottom of the 5 μm Gr. domain image shows a colourized image of the Gr. domains with similar crystal orientations located within a Cu grain.) (b) Polarized optical microscopy (POM) images of a Gr. sheet coated with LC mixture A on a glass substrate. The images show that the LC molecules were aligned along different azimuthal angles over each Gr. domain and along a uniaxial angle over the glass region. (c) POM images of the LC-coated Gr. films on the PDMS substrate after a complete growth process. LC molecules with different orientations on the Gr. domain exhibited a variety of birefringent colours. Some of the Gr. domains or copper grains are marked with small alphabet letters or underlined letters, respectively. Scale bars, 100 μm, and 10 μm for inset. Figure 1: Graphene domain size and LC alignment. ( a ) Scanning electron microscopy images of graphene (Gr.) synthesized through an incomplete growth process on a Cu foil, then transferred onto a glass substrate (The insets show magnified images of a single domain of Gr. The inset in the bottom of the 5 μm Gr. domain image shows a colourized image of the Gr. domains with similar crystal orientations located within a Cu grain.) ( b ) Polarized optical microscopy (POM) images of a Gr. sheet coated with LC mixture A on a glass substrate. The images show that the LC molecules were aligned along different azimuthal angles over each Gr. domain and along a uniaxial angle over the glass region. ( c ) POM images of the LC-coated Gr. films on the PDMS substrate after a complete growth process. LC molecules with different orientations on the Gr. domain exhibited a variety of birefringent colours. Some of the Gr. domains or copper grains are marked with small alphabet letters or underlined letters, respectively. Scale bars, 100 μm, and 10 μm for inset. Full size image Figure 1c shows optical images of an LC layer aligned on a Gr. sheet transferred to a PDMS substrate after complete film growth. Polarized optical microscopy images showed that different spatial geometries were associated with the different Gr. domain sizes. The LC layers on the 5 μm Gr. domains formed patterns with a domain size in the range of 50–100 μm, much larger than the 5 μm Gr. domain size. This trend was also observed in images shown in Fig. 1b and in Supplementary Fig. 7a , both of which captured images of incompletely grown Gr. films. Interestingly, the sizes and shapes of the LC alignment pattern corresponded not to the shape of the Gr. domain, but to the shape of the underlying Cu grain 50–100 μm in size. The same trend was observed in Gr. films with domain sizes of less than 30 μm ( Supplementary Fig. 12 ). Gr. domains in the range 5–30 μm tended to grow within the Cu grains without moving far over the Cu grain boundaries. As a result, the size distributions and orientations of the small Gr. domains within a Cu grain clearly identified the Cu grain boundaries in the image (the inset of Fig. 1a : 5 μm Gr. domain and Supplementary Figs 3d,13 and Note 4 ). The Gr. domains displayed a preferred growth orientation and growth rate, depending on the crystal orientations of the underlying Cu grain [27] , [28] , [29] , [30] . A group of graphene domains on a particular Cu grain yielded a mean anisotropic direction that reflected the nature of the Cu grains. Low-magnification birefringence optical images indicated that the LCs were overall aligned along the Cu grains, although the LCs on each Gr. domain were slightly elastically distorted by the preferred orientation, which differed from the mean direction of each Gr. domain, as indicated in the uneven colour within a single Cu grain ( Fig. 1c : 5 μm Gr. domain, also see Supplementary Fig. 7a ). By contrast, Gr. with domain sizes of 40 μm and 100 μm induced the LCs to clearly align along the Gr. domains, similar to the results observed among the disconnected domains ( Fig. 1b ). Unlike the growth of small-domain Gr., Gr. sheets with large domains formed across the Cu grain boundaries. As a result, the LCs aligned themselves according to the distribution of Gr. domains without relation to the Cu grain distribution (the inset of Fig 1b,c ). This result revealed that the LCs could be uniformly aligned along a Gr. domain due to strong interactions between the Gr. domains and the LC molecules. Large Gr. domains grew continuously across the Cu grain boundaries because during the initial growth stages, a smaller number of nuclei formed on the Cu grains ( Supplementary Fig. 4 ). The subsequent domain growth was much more strongly influenced by the orientation of the initial seed than by the crystal structure of the underlying Cu substrate. On the other hand, small Gr. domains grew from many nuclei and generally could not overcome the barrier presented by the Cu boundary. Although the birefringence images of the 40 and 100 μm domains differed from those of the 5–30 μm domains, these differences resulted not from different mechanisms of LC alignment, but rather from the growth mechanisms of underlying Gr. domain growth on the Cu surfaces ( Supplementary Note 5 ). A more detailed study of the origin of anisotropic anchoring between the Gr. layer and the LC is required to expand our understanding of this phenomenon. Direct observation of defects in graphene The LC mixture used in our experiments was composed of various molecules that formed a nematic phase. The composition ratio of the LC mixture could be used to adjust the phase transitions of the LC for the rapid detection of actual ruptures or nanoscale crack initiation in a Gr. sheet under external strain. A single-component LC, such as 4-cyano-4′-pentylbiphenyl, does not exhibit phase transition behaviour because there is no change in composition ( Supplementary Fig. 14 ). PDMS, which contains many pores and displays certain hydrophobic characteristics, can absorb small hydrophobic molecules [31] and displays molecule-specific absorption affinities ( Supplementary Fig. 15 ) [32] . A droplet of an LC mixture placed on a PDMS substrate underwent a concentration shift over time, in which the concentration of large polar molecules increased over time, causing a transition to a smectic (or crystal) phase in the LC mixture above a certain concentration. 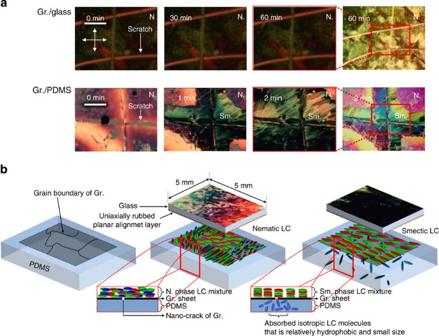Figure 2: LC phases on the graphene/PDMS substrates. (a) POM image of an LC phase transition on a graphene (Gr.) sheet suspended on glass and PDMS. The samples were cruciformly blemished with a razor blade before LC mixture A coating. Beginning from the scratched region, the nematic phase converted to a smectic (or crystal) phase on the artificially scratched Gr./PDMS substrate but not on the Gr./glass substrate. The orientations of the cross polarizers are indicated by the crossed arrows. Scale bars, 250 μm (b) Schematic representation of the phase transition on a Gr./PDMS substrate. The nematic phase (N.) was converted to a smectic (or crystal) phase (Sm.) by varying the composition of the LC mixture. Figure 2a shows the phase transition of the LC on a cruciformly blemished Gr. surface printed onto glass or PDMS. The sheets were intentionally scratched after wet transfer to the substrate and before LC mixture coating. The Gr./glass substrate without absorbed molecules did not display a change in the LC phase. The nematic LC on the Gr./PDMS substrate changed to a smectic (or crystal) LC in a cruciform pattern over time. This phenomenon occurred because the composition ratio of the LC molecules varied as certain molecules were absorbed into the PDMS substrate through lacerations in the Gr.. This behaviour can be used to observe the distribution of unavoidable defects, such as pinholes and cracks, that form in Gr. sheets during CVD synthesis and transfer processes [4] , [5] , [6] , [7] , [8] , [11] , [12] . If these defects are larger than the size of the molecules of the LC mixtures, the small hydrophobic molecules would be readily absorbed into the PDMS substrate through the defects, similar to the absorption through the intentional scratches introduced onto the Gr. sheets. The phase transitions of the LCs on the Gr./PDMS readily indicated the presence of nano-cracks and pinholes in the Gr. sheets, as shown in the schematic diagrams in Fig. 2b . Figure 2: LC phases on the graphene/PDMS substrates. ( a ) POM image of an LC phase transition on a graphene (Gr.) sheet suspended on glass and PDMS. The samples were cruciformly blemished with a razor blade before LC mixture A coating. Beginning from the scratched region, the nematic phase converted to a smectic (or crystal) phase on the artificially scratched Gr./PDMS substrate but not on the Gr./glass substrate. The orientations of the cross polarizers are indicated by the crossed arrows. Scale bars, 250 μm ( b ) Schematic representation of the phase transition on a Gr./PDMS substrate. The nematic phase (N.) was converted to a smectic (or crystal) phase (Sm.) by varying the composition of the LC mixture. 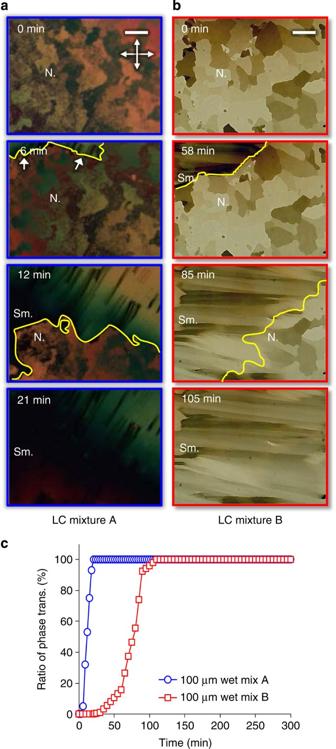Figure 3: POM image of the LC phase transition. The phase transition (trans.) ratios as a function of time for (a) LC mixture A, and (b) LC mixture B on Gr. sheets with 100 μm domains and wet-transferred onto a PDMS substrate. The orientations of the cross polarizers are indicated by the crossed arrows. Scale bars, 100 μm (c) Quantification of the defects in Gr. N., nematic phase; Sm., smectic phase. Full size image Figure 3 shows optical images of two types of LC mixtures on a PDMS substrate covered with a wet-transferred Gr. sheet with domain sizes of 100 μm. The velocity of the phase transition due to the selective molecular absorption of PDMS was proportional to the number of defects present and depended on the composition of the LC mixture. Figure 3a,b show the differences in the transition velocities of the mixtures A and B ( Supplementary Fig. 16 ) due to different composition and kinds of molecules. Gas chromatography–mass spectrometry measurements revealed that mixture A is composed of four kinds of molecules with relatively light molecular weight, whereas mixture B is composed of nine kinds of molecules with relatively heavy weight and wide weight distribution ( Supplementary Fig. 15 ). Figure 3: POM image of the LC phase transition. The phase transition (trans.) ratios as a function of time for ( a ) LC mixture A, and ( b ) LC mixture B on Gr. sheets with 100 μm domains and wet-transferred onto a PDMS substrate. The orientations of the cross polarizers are indicated by the crossed arrows. Scale bars, 100 μm ( c ) Quantification of the defects in Gr. N., nematic phase; Sm., smectic phase. Full size image The speed of the phase transition was calculated from the area ratio of the phase transition, as shown in Fig. 3c (see Supplementary Fig. 17 for a description of the calculation method). Mixture A exhibited a rapid phase transition from a nematic to a smectic (or crystal) phase. The area of the new smectic (or crystal) phase gradually increased over time. Mixture B resulted in a relatively slow phase change on PDMS and, as a result, displayed a distinct starting region for the transition within a Gr. sheet. This phase transition region facilitated the identification of relatively large defects. In the case of small defects, a phase transition could reflect the overall density of defects, rather than revealing the positions of the defects, owing to the nature of the second order transition accompanying the super-cooling and propagating boundary. The defect distributions on the Gr. sheets prepared with different domain sizes were quantitatively analysed by observing the phase transition of mixture B on three wet-transferred sheets. Interestingly, as the domain size increased, the speed of the transition in the mixture tended to increase ( Fig. 4a and Supplementary Fig. 16d–f ), even though the Gr. sample with smaller domains was expected to include a large number of domain boundaries that could easily generate defects. Unlike the Gr. sheet having 100 μm domains, the sheet having 5 μm domains displayed a slow transition after retardation over 100 min. Recently, Park et al. reported that Gr. sheets with small domains exhibited a better electrical performance than Gr. sheets with larger domains, in contrast with previous reports [33] . They suggested that this observation resulted from the presence of two different types of interconnections between neighbouring domains. Small domains tended to form strong primary connections involving covalent bonds. By contrast, large domains created relatively weak secondary connections in addition to the primary covalent bonds due to the overlap between the domains. The weak secondary connections increased the contact resistance. A similar interpretation could be applied to defect generation in Gr. As shown in the magnified scanning electron microscopy images and Raman spectra of Supplementary Figs 3,5, and 18 , Gr. sheets with domain sizes of 40 or 100 μm clearly displayed dark lines and a G/2D peak ratio composed of a bilayer between adjacent Gr. domains, unlike the sheets having 5 μm domains. These dark lines were thought to indicate the formation of domain overlap during CVD growth. Gr. sheets with small grains formed strongly connected domain boundaries that could prevent crack creation more effectively than large domains that were weakly connected by overlapping regions. The small molecules of an LC may not be able to penetrate through the small cracks in the domain boundaries. 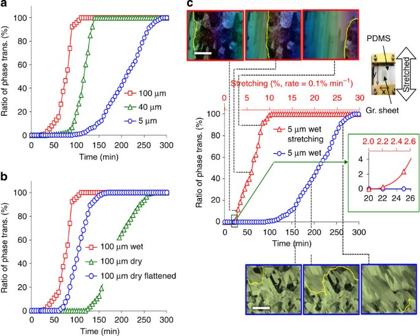Figure 4: Phase transition ratios versus time for the LC mixture B. (a) On Gr. sheets with various domain sizes, or (b) transferred using different transfer methods. (c) The variations in the phase transition (trans.) ratio on the Gr./PDMS substrate during stretching of the Gr./PDMS substrate (red triangle) or in the absence of stretching (blue circle), and POM images of the LC phase transition. Scale bars, 200 μm. Figure 4: Phase transition ratios versus time for the LC mixture B. ( a ) On Gr. sheets with various domain sizes, or ( b ) transferred using different transfer methods. ( c ) The variations in the phase transition (trans.) ratio on the Gr./PDMS substrate during stretching of the Gr./PDMS substrate (red triangle) or in the absence of stretching (blue circle), and POM images of the LC phase transition. Scale bars, 200 μm. Full size image After CVD growth, Gr. sheets must be transferred from the Cu foil onto a useful foreign substrate for device fabrication. The most common wet transfer method used for transferring small-area Gr. requires several steps, including the formation of a thin polymer film coating the Gr. sheet, printing onto a target substrate after Cu etching in chemical solvents, and the removal of the top polymer film from the Gr. [11] , [12] . These complicated steps can generate cracks in the Gr. The number of defects created by this wet transfer process was evaluated by preparing two dry transferred samples to permit a comparison with the wet-transferred sample. One dry sample was produced by etching the Cu foil gently after pouring and curing a PDMS solution over the Gr./Cu foil. The other dry sample was prepared by curing a PDMS layer directly after flattening the Gr./Cu foils using a roller. Figure 4b shows the phase transition speeds of the LC mixture B, observed for each of the three samples having domain sizes of 100 μm. The sample produced by wet transfer, which increased the probability of crack creation, exhibited the fastest transition speed, whereas the sample prepared by dry transfer underwent a slow change after retardation over 125 min because it contained a smaller number of defects. The sample that underwent a flattening process exhibited behaviour similar to that observed in the wet-transfer sample. Flattening via mechanical rolling appeared to generate additional cracks in the Gr. sheet. Crack generation in Gr. under an external strain The phase transitions in the LCs due to cracks in Gr. created under external strain were examined. Although the theoretical calculations of Ruoff et al. reported that polycrystalline Gr. begins to form cracks at the domain boundaries under an external strain of 7–10% (ref. 15 ). Experimentally, polycrystalline Gr. sheets with pinholes and nano-cracks may be broken under much smaller strains. The calculation of Ruoff et al. did not consider the presence of any defects in the Gr. sheet other than those associated with the domain boundaries [15] . Figure 4c shows the rapid evolution of crack generation in Gr. under an external strain. The phase transition of the LC mixture B on a Gr. sheet having 5 μm domains and mounted on PDMS was continuously measured at a strain of 0.1% min −1 (see Supplementary Figs 16g–h, 19 and Movie for mixture A). Without external strain, the Gr. exhibited a slow phase transition from a nematic to a smectic (or crystal) phase after retardation for 100 min at the pinholes or cracks created by the growth and wet-transfer processes. Alternatively, the application of an external strain of 2.20% resulted in a rapid phase transition in the LC due to the creation of new cracks and an increase in the crack or pinhole size due to the strain. This result corresponded to the electrical measurement results, in which the resistance of a Gr. sheet increased suddenly in response to a 2.18% strain ( Supplementary Fig. 20 and Note 6 ). The polydomain distributions in Gr. sheets grown by CVD methods were observed on the basis of the alignment of LC molecules over an underlying Gr. domain due to an anchoring force. Optical images of the birefringence of the LC alignment depended on the Gr. domain size. Small Gr. domains (5 μm in size) formed with a preferred growth orientation and were confined to the boundaries of the underlying Cu grains. As a result, a low-magnification birefringence optical image reflected the shape of the underlying Cu grain on the basis of the mean anisotropic direction of the grain shape. In addition, we observed that small hydrophobic molecules in the LC mixture were effectively absorbed into the PDMS substrates. This absorption process may be useful for quantifying defects in a Gr. sheet synthesized by CVD or for rapidly visualizing crack creation in a Gr. sheet under an external strain. This simple method for observing the defect generation process and the domains in a Gr. sheet provides a promising route to evaluating the electrical and mechanical performances of Gr. for applications in flexible and stretchable electronics. Gr. synthesis and transfer Gr. sheets with different domain sizes were synthesized on a Cu foil (purity 99.8%) by controlling both the CH 4 flow rate and the H 2 annealing time to suppress the formation of Gr. nucleation seeds. The Cu foils were cleaned in acid and inserted into the tubular quartz tube of a CVD system under H 2 gas flow for 30 min before the growth process. During the growth step, the CH 4 :H 2 gases in a ratio of 8:20 sccm or 1:10 sccm were injected to induce Gr. growth with domain sizes of 5–20 μm or >30 μm, respectively (also see Supplementary Method ). The Cu foils were subsequently rapidly cooled to room temperature. The Gr. sheets were then transferred to a foreign substrate using a wet-etching method to remove Cu after applying a PMMA or PDMS thin polymer layer coating on the Gr./Cu foil. LC alignment Commercially available nematic LC mixtures A and B (A: JNC Chisso, IAN-5000XX T1, B: Merck, MLC-7026-000) were used here. These mixtures were composed of various molecules. The ‘A’ mixture displayed a positive dielectric anisotropy, whereas the ‘B’ mixture displayed a negative dielectric anisotropy. A 0.5 μl droplet of the LC mixture was dropped onto a Gr. substrate (2 × 2 cm), and another smaller glass substrate (5 × 5 mm) was coated with a uniaxially rubbed planar alignment layer (70 nm) or a vertical alignment layer placed over the LC drop. Although the cover substrate with a vertical alignment layer provided a clearer birefringence image compared with the parallel layer, it was difficult to clearly observe the domain boundaries at the start of the phase transition from nematic to smectic (or crystal) ( Supplementary Fig. 21 ). In addition, the LCs could become aligned in the absence of a rubbed alignment layer ( Supplementary Fig. 8 ). The fixed ratio of LC volume to cover glass size determined the exact thickness of the LC layer, which is needed for the quantitative analysis of defect numbers in the Gr. on the basis of the LC phase transition measurements. The initial LC layer thickness was approximately 20 μm. The LC alignment and texture were observed under cross polarizers using a polarizing microscope (Olympus, BX53, × 50– × 1000). The axis of the polarizer was adjusted to maximize the contrast among the LC domains. How to cite this article: Son, J.-H. et al. Detection of graphene domains and defects using liquid crystals. Nat. Commun. 5:3484 doi: 10.1038/ncomms4484 (2014).